MyD88 signalling in colonic mononuclear phagocytes drives colitis in IL-10-deficient mice Commensal bacterial sensing by Toll-like receptors is critical for maintaining intestinal homeostasis, but can lead to colitis in the absence of interleukin-10. Although Toll-like receptors are expressed in multiple cell types in the colon, the cell type(s) responsible for the development of colitis are currently unknown. Here we generated mice that are selectively deficient in MyD88 in various cellular compartments in an interleukin-10 −/− setting. Although epithelial expression of MyD88 was dispensable, MyD88 expression in the mononuclear phagocyte compartment was required for colitis development. Specifically, phenotypically distinct populations of colonic mononuclear phagocytes expressed high levels of interleukin-1β, interleukin-23 and interleukin-6, and promoted T-helper 17 responses in the absence of interleukin-10. Thus, gut bacterial sensing through MyD88 in mononuclear phagocytes drives inflammatory bowel disease when unopposed by interleukin-10. Increasing evidence supports the notion that inflammatory bowel disease (IBD) results from a dysregulated interaction between the host immune system and its commensal microbiota [1] . Commensal bacteria are most abundant in the colon and they normally co-exist with the host in a mutually beneficial relationship. At the same time, the mammalian host must maintain the ability to recognize pathogenic microbes in the colon and respond appropriately to contain and eliminate them. Although the exact mechanism by which commensal bacteria and pathogenic bacteria are distinguished is unclear, recent evidence indicates that multiple mechanisms exist to limit inflammatory immune responses against commensal microbes. One such mechanism involves secretion of interleukin (IL)-10 in the intestinal mucosa. In the absence of IL-10, mice develop severe colitis with variable kinetics, depending on the facility [2] , [3] . MyD88 deficiency completely rescues colitis in IL-10 −/− mice [4] . However, the cell types responsible for inducing colitogenic signals in IL-10 −/− mice remain unknown. Both haematopoietic and non-haematopoietic cell types express MyD88. In the intestinal mucosa, enterocytes express MyD88 and respond to a variety of Toll-like receptor (TLR) ligands [5] . Transgenic expression of MyD88 by Paneth cells in MyD88 −/− mice is sufficient to induce anti-microbial peptides upon sensing of commensal bacteria and prevents bacterial translocation [6] . Another important cell type that recognizes bacteria through the TLR–MyD88 pathway is the mononuclear phagocyte (MNP), consisting of macrophages and dendritic cells (DCs). The colonic lamina propria contains distinct macrophages and DC populations, with partially overlapping phenotypic and functional properties [7] , [8] . The colonic MNPs can be divided into macrophages that are CX 3 CR1 + CD11b + , and DCs that contain the CD103 + CD11b − , CD103 + CD11b + and CD103 − CD11b + subsets [9] . Colonic macrophages contain at least two subsets, CD11c + and CD11c − , and are both considered to be anti-inflammatory, as they predominantly secrete IL-10, but not IL-12 or tumour necrosis factor-α, and suppress inflammatory responses [9] , [10] , [11] , [12] . Under inflammatory conditions in a T-cell-mediated colitis model, monocyte-derived E-cadherin + CD103 − DCs predominate the colon and secrete colitogenic cytokines such as IL-23 and IL-6 (refs 9 , 13 ). However, very little is known about the role of specific MNP subsets in chronic spontaneous colitis that arise in the absence of IL-10. To interrogate the cell types responsible for mediating spontaneous colitis that arises in IL-10-deficient mice, we generated mice that are selectively deficient in MyD88 in various cellular compartments and followed colitis progression over time. We further characterized the phenotype and function of MNPs in which MyD88-dependent signals drive IBD in IL-10 −/− mice. Our results reveal the selective importance of gut bacterial sensing by MNPs through the MyD88-dependent pathway in mediating IBD and place the colonic MNPs as the key initiator of colitogenic inflammation. Cell-type-specific MyD88 function in colitis development IL-10 −/− mice develop spontaneous colitis around 4–8 weeks of age in our facility, which depends on intestinal bacteria sensing through MyD88-dependent signals [4] . We first tested the existence of Helicobacter spp ., which is known to drive colitis development in IL-10-deficient mice. Mice were screened by PCR and 16S ribosomal RNA sequences, and H. typhlonicus , H. hepaticus , H. ganmani and H. rodentium were detected in our colony (data not shown). To confirm that colitis is induced by commensal bacteria, we treated IL-10 −/− mice with antibiotics, and indeed pathology measured by endoscopic colitis score, histopathologic score and mesenteric lymph nodes (MLNs) enlargement were all reversed after 2 weeks of treatment ( Supplementary Fig. S1 ). To determine the cell types responsible for colitis development in IL-10 −/− mice, mice deficient in MyD88 expression in various cell types were generated. Mice carrying MyD88 floxed allele(s) were crossed to an IL-10 −/− background, and was further crossed to different Cre-recombinase-expressing mouse lines; for example, MyD88 FL , Villin–Cre(+), IL-10 −/− (Villin–MyD88/IL-10 knock out (KO), targeting MyD88 deletion in intestinal epithelial cells); MyD88 FL , CD11c–Cre(+), IL-10 −/− (CD11c–MyD88/IL-10 KO, targeting DCs [14] ); and MyD88 FL , LysM–Cre(+), IL-10 −/− (LysM–MyD88/IL-10 KO, targeting phagocytes). The deletion efficacy in the respective cell types was found to be 100, 99 and 83% respectively ( Supplementary Fig. S2a–d ). As expected, over 91% of IL-10 −/− mice showed severe inflammation and an increase in the number of MLN cells by 15 weeks of age ( Fig. 1 ). Macroscopically, Villin–MyD88/IL-10 KO mice showed signs of colitis comparable to IL-10 −/− mice, including intestinal wall thickening, unformed stools and MLN hypertrophy. In contrast, minimal signs of inflammation were detected in either CD11c–MyD88/IL-10 KO or LysM–MyD88/IL-10 KO mice ( Fig. 1a ). In addition, histological examination detected pathological changes, including epithelial hyperplasia and massive leukocytic infiltration, only in the tissue of IL10 −/− and Villin–MyD88/IL-10 KO mice, but not in CD11c–MyD88/IL-10 KO or LysM–MyD88/IL-10 KO mice ( Fig. 1b ). Consistently, MLN hypertrophies was detected in IL-10 −/− mice and in Villin–MyD88/IL-10 KO mice, but cell numbers in the MLN were only slightly above the wild-type (WT) control in CD11c–MyD88/IL-10 KO or LysM–MyD88/IL-10 KO mice ( Fig. 1c ). Taken together, these data indicated that MyD88 signals in CD11c + and LysM + cells, but not in epithelial cells, are required for the onset of colitis in the absence of IL-10. 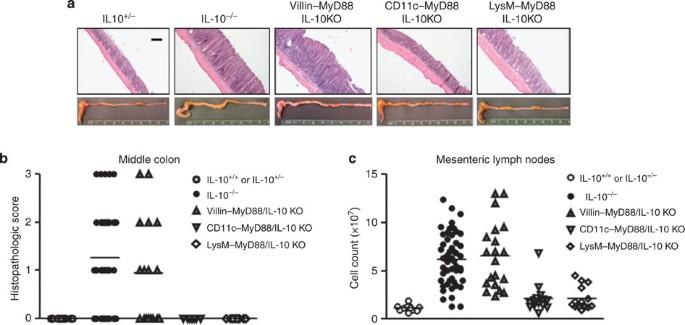Figure 1: Cell type-specific MyD88 deletion in IL-10−/−colitis. (a) Haematoxylin and eosin staining in middle colon tissue and photograph of presentative colon of 15 weeks old mice. Scale bar, 200 μm. (b) Histopathological score using middle colon of IL-10+/+or IL10+/−(n=15; age raging 10–15 weeks old), IL-10−/−(n=32; age raging 9–18 weeks old), Villin–MyD88/IL-10 KO (n=16; 9–15 weeks old), CD11c–MyD88/IL10-KO (n=6; age raging 15–18 weeks old) and LysM–MyD88/IL-10 KO mice (n=8; age raging 10–15 weeks old). Samples were collected only from sets of littermates for the comparison between control IL-10−/−and each conditional KO strains. (c) Cell number of mesenteric lymph nodes cells of IL-10+/+or IL10+/−(n=11), IL-10−/−(n=50), Villin–MyD88/IL-10 KO (n=20), CD11c–MyD88/IL10-KO (n=14) and LysM–MyD88/IL-10 KO mice (n=14) at 15 weeks old. Figure 1: Cell type-specific MyD88 deletion in IL-10 −/− colitis. ( a ) Haematoxylin and eosin staining in middle colon tissue and photograph of presentative colon of 15 weeks old mice. Scale bar, 200 μm. ( b ) Histopathological score using middle colon of IL-10 +/+ or IL10 +/− ( n =15; age raging 10–15 weeks old), IL-10 −/− ( n =32; age raging 9–18 weeks old), Villin–MyD88/IL-10 KO ( n =16; 9–15 weeks old), CD11c–MyD88/IL10-KO ( n =6; age raging 15–18 weeks old) and LysM–MyD88/IL-10 KO mice ( n =8; age raging 10–15 weeks old). Samples were collected only from sets of littermates for the comparison between control IL-10 −/− and each conditional KO strains. ( c ) Cell number of mesenteric lymph nodes cells of IL-10 +/+ or IL10 +/− ( n =11), IL-10 −/− ( n =50), Villin–MyD88/IL-10 KO ( n =20), CD11c–MyD88/IL10-KO ( n =14) and LysM–MyD88/IL-10 KO mice ( n =14) at 15 weeks old. Full size image MyD88 in colonic MNPs is required for cytokine responses As CD11c and LysM are expressed by antigen-presenting cells, such as DCs and macrophages, the absence of colitis seen in CD11c–MyD88/IL-10 KO and LysM–MyD88/IL-10 KO mice implicate the importance of these cell types in secreting proinflammatory cytokines and inducing colitogenic T-cell responses. To this end, we measured the secretion of IL-12 p40 from the supernatant of colon tissue explant cultures. IL-12 p40 is a cytokine subunit necessary to form intact IL-12 p70 and IL-23, which have a key role in T-helper (Th)1 and Th17 responses, respectively [15] , [16] , [17] , [18] , [19] . Colonic tissue explants from Villin–MyD88/IL-10 KO mice produced similar levels of IL-12 p40 as that produced by the control IL-10 −/− tissue ( Fig. 2a ). In contrast, colonic tissues taken from CD11c–MyD88/IL-10 KO and LysM-MyD88/IL-10 KO mice failed to secrete appreciable levels of IL-12 p40 ( Fig. 2a ). To extend this finding to other proinflammatory cytokines, we next measured the levels of IL-1β, IL-6 and tumour necrosis factor-α messenger RNA from colonic tissues by quantitative PCR. Again, mRNA levels of all of these cytokines were significantly reduced in the colons of CD11c–MyD88/IL-10 KO and LysM-MyD88/IL-10 KO mice compared with IL-10 −/− mice, whereas Villin–MyD88/IL-10 KO mice expressed similarly high levels of these cytokines as the IL-10 −/− controls ( Fig. 2b ). These results indicate that MNPs responsible for the onset of colitis rely on MyD88-dependent signals for the secretion of proinflammatory cytokines in the colon. 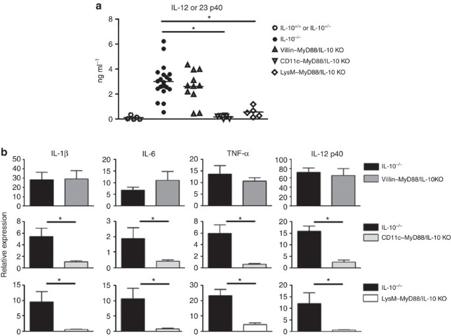Figure 2: Regulation of inflammatory cytokines in IL-10−/−mice. (a) ELISA analysis for IL-12/23 p40 level of colon explants cultures. IL-10+/+or IL10+/−(n=5), IL-10−/−(n=21), Villin–MyD88/IL-10 KO (n=11), CD11c–MyD88/IL10-KO (n=6) and LysM–MyD88/IL-10 KO mice (n=5) at 12–15 weeks old were used. (b) Relative mRNA expression levels in the colon tissue measured by quantitative PCR. At least six sets of littemates were used in each genotypes. Error bars represent mean±s.e.m.*P<0.05 (unpaired Student'st-t test). Figure 2: Regulation of inflammatory cytokines in IL-10 −/− mice. ( a ) ELISA analysis for IL-12/23 p40 level of colon explants cultures. IL-10 +/+ or IL10 +/− ( n =5), IL-10 −/− ( n =21), Villin–MyD88/IL-10 KO ( n =11), CD11c–MyD88/IL10-KO ( n =6) and LysM–MyD88/IL-10 KO mice ( n =5) at 12–15 weeks old were used. ( b ) Relative mRNA expression levels in the colon tissue measured by quantitative PCR. At least six sets of littemates were used in each genotypes. Error bars represent mean±s.e.m. *P <0.05 (unpaired Student's t -t test). Full size image MyD88 in colonic MNPs drives Th1 and Th17 expansion To determine the cellular mechanism of colonic inflammation in IL-10 −/− mice, we next examined the phenotype of CD4T cells in the lymph nodes draining the colon. Cytokine secretion from MLN T cells stimulated with anti-CD3 antibody indicated that although high levels of IL-17A and interferon (IFN)-γ are produced from MLN of IL-10 −/− and Villin–MyD88/IL-10 KO mice, these cytokines remained barely detectable in CD11c–MyD88/IL-10 KO and LysM-MyD88/IL-10 KO mice ( Fig. 3a ). We also tested the cytokine secretion from lamina propria T cells stimulated with anti-CD3 antibody; the result was similar to that of MLN cells ( Fig. 3b ). Accordingly, both IL-17A and IFN-γ mRNA levels were much lower in the colonic tissue from CD11c–MyD88/IL-10 KO and LysM–MyD88/IL-10 KO mice compared with IL-10 −/− control ( Fig. 3c ), indicating that such Th1/Th17 expansion occurred within the tissue only upon MyD88-dependent stimulation of MNPs. Although the lack of colitis development in CD11c–MyD88/IL-10 KO and LysM–MyD88/IL-10 KO mice was likely due to the absence of intestinal bacterial sensing in these mice, it was also possible that expansion of the Th2 and/or regulatory T cell (Treg) compartments may have contributed to protection from disease by inhibiting the colitogenic IL-17 and IFN-γ response. To address the latter possibility, mRNA levels of IL-4 and the frequency of Tregs in the colon were measured. There was no change in IL-4 levels ( Fig. 3c ) or the frequency of Treg cells in CD11c–MyD88/IL-10 KO and LysM–MyD88/IL-10 KO mice compared with IL-10 −/− control group ( Fig. 3d ). These data suggested that Th1 and Th17 expansion occurs in the colon and in the MLN of IL-10 −/− mice in a manner dependent on bacterial sensing by CD11c + and LysM + MNPs, without affecting the frequency of Th2 or Treg subsets. However, the suppressive function of Tregs is abrogated by the absence of IL-10 (refs 20 , 21 , 22 ). 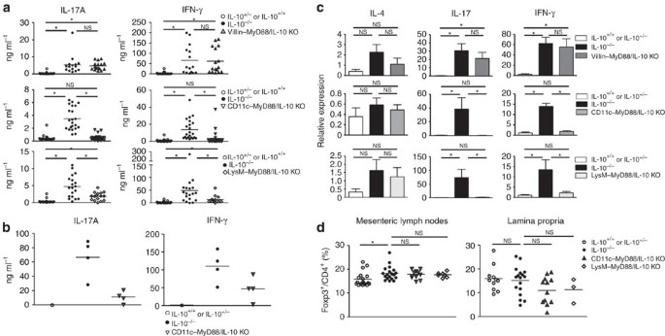Figure 3: Regulatory and effector T cells in IL-10−/−mice. (a) Mesenteric lymph nodes cells were cultured in the presence of plate-bound anti-CD3ε antibody for 48 h. IL-17A and IFN-γ levels in the culture supernatants were mesured by ELISA assays. Sets of littermates at 13–22 weeks old were used for the comparison between control IL-10−/−and each conditional KO strains. IL-10+/+or IL-10+/−mice were of same age range as IL-10−/−experimental mice (of which some mouse samples were shared among Villin–, CD11c– and LysM–Cre experiments). Each plot indicates individual mouse. Shown is the combined data of at least five repeated experiments. (b) Colonic lamina propria cells were cultured in the presence of plate-bound anti-CD3ε antibody for 48 h. IL-17A and IFN-γ levels in the culture superrnatants were mesured by ELISA assays. WT plot represents the pooled sample of three mice. Only sets of littermates were used for the comparison between control IL-10−/−(each plot represent individual mouse) and CD11c–MyD88/IL-10 KO mice (each plot is either individual mouse or pooled sample of two mice). (c) Relative mRNA expression levels of colon tissue measured by quantitative PCR. At least six sets of littermates at 13–17 weeks old were used. IL-10+/+or IL-10+/−mice samples (n=7) are shared among Villin–, CD11c– and LysM–Cre experiments. (d) Frequency of Foxp3+in MLNs and colonic lamina propria were analysed by flow cytometry. Each plot indicates an individual mouse. Error bars represent mean±s.e.m.*P<0.05 (unpaired Student'st-test). Figure 3: Regulatory and effector T cells in IL-10 −/− mice. ( a ) Mesenteric lymph nodes cells were cultured in the presence of plate-bound anti-CD3ε antibody for 48 h. IL-17A and IFN-γ levels in the culture supernatants were mesured by ELISA assays. Sets of littermates at 13–22 weeks old were used for the comparison between control IL-10 −/− and each conditional KO strains. IL-10 +/+ or IL-10 +/− mice were of same age range as IL-10 −/− experimental mice (of which some mouse samples were shared among Villin–, CD11c– and LysM–Cre experiments). Each plot indicates individual mouse. Shown is the combined data of at least five repeated experiments. ( b ) Colonic lamina propria cells were cultured in the presence of plate-bound anti-CD3ε antibody for 48 h. IL-17A and IFN-γ levels in the culture superrnatants were mesured by ELISA assays. WT plot represents the pooled sample of three mice. Only sets of littermates were used for the comparison between control IL-10 −/− (each plot represent individual mouse) and CD11c–MyD88/IL-10 KO mice (each plot is either individual mouse or pooled sample of two mice). ( c ) Relative mRNA expression levels of colon tissue measured by quantitative PCR. At least six sets of littermates at 13–17 weeks old were used. IL-10 +/+ or IL-10 +/− mice samples ( n =7) are shared among Villin–, CD11c– and LysM–Cre experiments. ( d ) Frequency of Foxp3 + in MLNs and colonic lamina propria were analysed by flow cytometry. Each plot indicates an individual mouse. Error bars represent mean±s.e.m. *P <0.05 (unpaired Student's t -test). Full size image Cell specificity of MyD88 deletion We next investigated the MNP cell types in which MyD88 is depleted in our conditional KO mice. Consistent with the previous studies of small intestine and colon MNPs [23] , [24] , [25] , [26] , [27] , we detected two major CD11c + populations, CD11c + CD11b − (P1) and CD11c + CD11b + (P2). The CD11c − CD11b + population consisted of two separate groups, CD11c − CD11b + side scatter (SSC) lo Siglec-F − macrophages (P3) and CD11c − CD11b + SSC hi Siglec-F + eosinophils ( Fig. 4a ). Representative Diff-Quick staining of cytospin preparations revealed that although P1 and P3 were morphologically homogeneous, P2 population was morphologically heterogeneous. Analysis of cell surface markers ( Fig. 4b ) indicated that P1 is CD103 + CX3CR1 − DEC205 + F4/80 − , corresponding to the DC4 population found in isolated lymphoid follicles in the colon [9] . The P3 expression profile (DEC205 − F4/80 + CX3CR1 + CD103 − F4/80 + CD11b + ) is consistent with the MP1 (CD11c − macrophages) that are distributed in the lamina propria of the mouse colon [9] . As observed from the heterogeneous morphology ( Fig. 4a ), the P2 population consisted of three separate cell types as follows: (1) CD103 − CD11b + CD11c + DCs (DC3 CD103 − ); (2) CD103 + CD11b + CD11c + DCs (DC3 CD103 + ); and (3) CD11c + CD103 − CX3CR1 + macrophages (MP2; Supplementary Fig. S3 ) [9] . To investigate which cell populations are targeted by CD11c–Cre and LysM–Cre transgene expression, we crossed these Cre-recombinase-expressing alleles to Rosa26-STOP FL -EYFP reporter mice [28] . As expected, CD11c–Cre was highly expressed in the CD11c + population MNPs represented by P1 and P2 subsets. In contrast, LysM–Cre was expressed primarily in P2 and P3 subsets. Of note, neither CD11c–Cre nor LysM–Cre was expressed by P4 cells, excluding the possibility of eosinophils being responsible for colitis development in IL-10 −/− hosts. Expression of LysM, a myeloid cell marker, in P2 and P3 populations is consistent with the fact that the P2 population consists of the CX3CR1 + CD11c + MP2 cells, which are of monocyte origin [24] , [25] , and P3 representing the MP1 macrophages ( Fig. 4b,c ). These data suggest that although P1 and P3 may contribute to colitogenesis in IL-10 −/− mice, the expression of MyD88 in P1 (in LysM–MyD88/IL-10 KO mice) or P3 (in CD11c–MyD88/IL-10 KO mice) is not sufficient to drive colitis in the respective mouse lines. Therefore, the key colitogenic potential appears to rest with the MNP populations within the P2 group of cells. 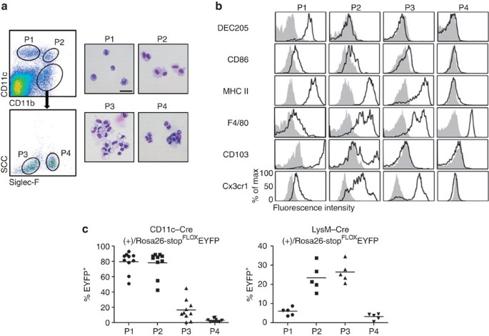Figure 4: Analysis of MyD88 deletion specificity. (a) Four subsets of colonic lamina propria cells separated using CD11b, CD11c, Siglec-F and SSC. Pictures are Diff-Quick staining of each of sorted subsets. Scale bar, 20 μm. (b) Cell surface phenotype of four populations. Filled histograms are the isotype control. (c) Frequency of EYFP+cells in the colonic lamina propria of CD11c–Cre(+)/Rosa26-STOPFLEYFP (n=10) and LysM–Cre(+)/Rosa26-STOPFLEYFP (n=5). Figure 4: Analysis of MyD88 deletion specificity. ( a ) Four subsets of colonic lamina propria cells separated using CD11b, CD11c, Siglec-F and SSC. Pictures are Diff-Quick staining of each of sorted subsets. Scale bar, 20 μm. ( b ) Cell surface phenotype of four populations. Filled histograms are the isotype control. ( c ) Frequency of EYFP + cells in the colonic lamina propria of CD11c–Cre(+)/Rosa26-STOP FL EYFP ( n =10) and LysM–Cre(+)/Rosa26-STOP FL EYFP ( n =5). Full size image Proinflammatory role of colonic CD11b + CD11c + cells To characterize the functional relevance of P1–P3 populations, we first sorted the P1–P3 MNP subsets from IL-10 sufficient (WT) non-colitic mice and examined their relative expression levels for TLRs and cytokine genes by quantitative PCR at a steady state ( Fig. 5 ). The P2 population expressed a wide range of TLRs and proinflammatory cytokine mRNA, including IL-1β, IL-6 and IL-23 p19, which are important for Th17 cell differentiation and expansion [27] , [29] , [30] , [31] . Moreover, the P2 cells expressed the highest level of IL-10 at steady state. In addition, P3 expressed several TLRs and moderately expressed cytokines, including IL-1β and IL-6. In contrast, P1 cells had minimal expression of TLRs or cytokines, except for TLR9. Importantly, all subsets expressed comparable levels of MyD88. These data suggest that P2 contains both immunoregulatory IL-10-secreting cells and cells capable of responding to various TLR ligands and secreting innate proinflammatory cytokines that can skew naive CD4T cells to the Th17 phenotype. 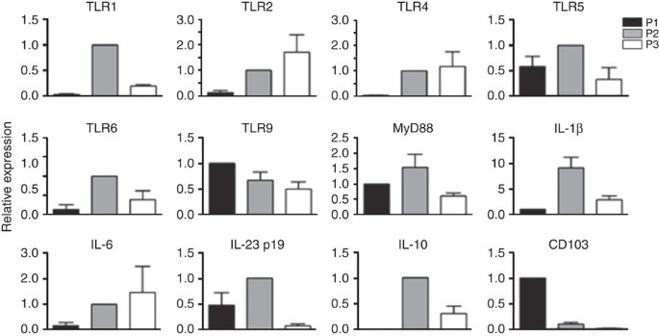Figure 5: Expression of TLRs and cytokines by P2 population. P1–P3 populations were sorted from pooled colon sample of over 10 B6 mice. mRNA levels were measured by quantitative PCR. Combined data from two to four independent experiments is shown. Error bars represent mean±s.e.m. Figure 5: Expression of TLRs and cytokines by P2 population. P1–P3 populations were sorted from pooled colon sample of over 10 B6 mice. mRNA levels were measured by quantitative PCR. Combined data from two to four independent experiments is shown. Error bars represent mean±s.e.m. Full size image CCR2 deficiency does not reverse colitis in IL-10 −/− mice Results thus far suggest that the P2 population contains cells capable of inducing colitis development in IL-10 −/− mice upon microbial sensing upstream of MyD88. To determine the MNP constituency in IL-10 −/− colitic mice, we examined surface phenotype of MNPs from colitic IL-10 −/− mice. Compared with non-colitic IL-10 +/− mice, P2 cells were slightly increased in number and the MP2 CX3CR1 + subset increased in frequency in IL-10 −/− mice ( Fig. 6a,b ; Supplementary Fig. S4 ), suggesting that the MP2 CX3CR1 + subset may be responsible for colitis phenotype in IL-10-deficient mice. We also found that the CD11c − CD11b + cells with very low SSC were predominant in the inflamed colon of IL-10 −/− mice ( Fig. 6a,b ). Furthermore, this inflammation-dependent P3 population expressed higher levels of Gr-1 and lower levels of CX3CR1 than the P3 population from the non-colitic IL-10 +/− mice ( Fig. 6a ), suggesting that they are derived from inflammatory monocytes [32] . Previous studies in the T-cell transfer colitis model reported the recruitment of inflammatory monocytes that secrete Th17-inducing cytokines [9] , [13] . Further, C–C chemokine receptor type 2 (CCR2)-dependent migration of inflammatory monocytes is critical for the pathogenesis of dextran sulphate sodium-induced colitis [33] . To test whether CCR2-dependent migration of MNPs is required for colitis development in IL-10 −/− mice, IL-10 −/− mice were crossed to CCR2 −/− mice to generate IL-10 −/− CCR2 −/− double KO mice. Spontaneous colitis that develops in IL-10 −/− mice was not reversed by CCR2 deficiency based on multiple parameters, including the severity and kinetics of colitis disease, and the Th17 or Th1 responses in the MLNs ( Supplementary Fig. S5 ). This prompted us to examine the MNP subsets in the colitic colon of CCR2 −/− IL-10 −/− mice. There was no significant difference in the overall frequencies of P1 or P3 MNPs in the inflamed colons of CCR2 −/− IL-10 −/− mice compared with IL-10 −/− mice. These data indicated that inflammatory monocytes have CCR2-independent redundant mechanisms of migration, and CCR2 deficiency is not sufficient to reverse the colitis in IL-10 −/− mice. 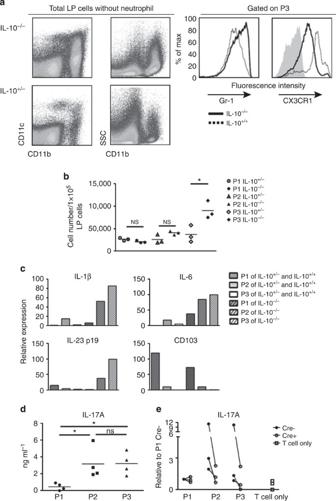Figure 6: P2 and P3 populations and Th17 induction. (a) Flow cytometry analysis. Filled histogram in CX3CR1 panel is the negative control using CX3CR1+/+/IL-10+/+mice. (b) Cell numbers of P1–P3 populations per 1.0×105of total colonic lamina propria cells were calculated using flow cytometry data. Each plot indicates an individual mouse.*P<0.05 (unpaired Student'st-test). (c) P1–P3 populations from pooled colon samples of IL-10-sufficient mice and colitic IL10−/−were sorted, and relative mRNA expression levels were measured by quantitative PCR. Data shown are respresentative of two independent experiments with similar result. (d) P1–P3 populations sorted from colitic IL10−/−mice were co-cultured with naive CD4T cells in the presence of anti-CD3ε antibody. Culture supernatants were used to measure IL-17A by ELISA assay. Data shown is a total of four independent experiments.*P<0.05 (unpaired Student'st-test). (e) P1–P3 population sorted from pooled colon samples of control IL-10−/−and CD11c–MyD88/IL-10 KO mice were co-cultured with naive CD4T cells in the presence of anti-CD3ε antibody. Culture supernatants were used to measure IL-17A by ELISA assay. Each value was normalized to that of P1(Cre−) sample. Data shown are the total of three independent experiments. Figure 6: P2 and P3 populations and Th17 induction. ( a ) Flow cytometry analysis. Filled histogram in CX3CR1 panel is the negative control using CX3CR1 +/+ /IL-10 +/+ mice. ( b ) Cell numbers of P1–P3 populations per 1.0×10 5 of total colonic lamina propria cells were calculated using flow cytometry data. Each plot indicates an individual mouse. *P <0.05 (unpaired Student's t -test). ( c ) P1–P3 populations from pooled colon samples of IL-10-sufficient mice and colitic IL10 −/− were sorted, and relative mRNA expression levels were measured by quantitative PCR. Data shown are respresentative of two independent experiments with similar result. ( d ) P1–P3 populations sorted from colitic IL10 −/− mice were co-cultured with naive CD4T cells in the presence of anti-CD3ε antibody. Culture supernatants were used to measure IL-17A by ELISA assay. Data shown is a total of four independent experiments. *P <0.05 (unpaired Student's t -test). ( e ) P1–P3 population sorted from pooled colon samples of control IL-10 −/− and CD11c–MyD88/IL-10 KO mice were co-cultured with naive CD4T cells in the presence of anti-CD3ε antibody. Culture supernatants were used to measure IL-17A by ELISA assay. Each value was normalized to that of P1(Cre−) sample. Data shown are the total of three independent experiments. Full size image MyD88 in CD11c + CD11b + cells amplifies colonic inflammation Th17 cells have a key pathogenic role in colitis that develops in IL-10 −/− mice, indicated by the fact that colitis develops in IL-12 p35 −/− /IL-10 −/− mice, but not in IL-12 p40 −/− /IL-10 −/− nor IL-23 p19 −/− /IL-10 −/− mice [17] . To determine which of the MNP subsets are involved in Th17 differentiation in the colon of IL-10 −/− mice, P1–P3 populations were sorted from IL-10 −/− colitic mice, and cytokine mRNA expression was analysed. Of note, not only the P2 but also the P3 population showed high levels of Th17 skewing cytokines, including IL-1β, IL-23 p19 and IL-6 in the inflamed colon ( Fig. 6c ). To test the ability of these cell populations to support Th17 differentiation, sorted P1–P3 populations from IL-10 −/− mice were co-cultured with naive splenic CD4T cells, and IL-17A secretion was measured from the supernatant upon anti-CD3 antibody stimulation. Consistent with the mRNA profile, both P2 and P3, but not P1, populations induced robust IL-17A secretion from CD4T cells ( Fig. 6d ). Further, to examine whether the Th17-inducing phenotype of MNPs in IL-10 −/− mice indeed depends on MyD88 expression by the respective MNP populations, we sorted MNP subsets from CD11c–MyD88/IL-10 KO and control IL-10 −/− mice and co-cultured these cells with naive splenic CD4T cells. Importantly, in the absence of MyD88 expression in the CD11c + MNP subsets, neither P2 nor P3 MNP subsets supported IL-17A production from naive CD4T cells ( Fig. 6e ). These data suggested that the P2 population initiates colonic inflammation through bacterial sensing via MyD88, and subsequently recruits inflammatory macrophages to the tissue. Together, P2 and inflammatory macrophages in the P3 gate support the induction of colitogenic Th17 cells in situ in the absence of IL-10. The TLR–MyD88 signalling pathway, which is engaged upon commensal microbiota recognition, has an important role in maintaining intestinal homeostasis [34] . In the absence of the key suppressive cytokine IL-10, MyD88-dependent signals lead to inflammation and colitis [4] . In this study, we examined the cell types responsible for inducing colitis in IL-10 −/− hosts. Our data revealed that MyD88 deletion in intestinal epithelial cells did not affect colitis progression in IL-10 −/− mice. However, deletion of MyD88 in CD11c + or LysM + MNPs led to a near complete abrogation of colitis in IL-10 −/− hosts. Further analyses showed that CD11c + CD11b + cell compartment contain cells that likely act as initiators of colitis through the secretion of proinflammatory cytokines, which are normally suppressed by IL-10. Our results are consistent with previous report demonstrating that myeloid-specific deletion of Stat3—a key intermediate of IL-10 signalling—develop colitis that can be prevented by TLR4 deficiency [35] . Helicobacter spp . are known to drive colitis in IL-10-deficient mice [36] , [37] and are present in our colony. Therefore, we speculate that MyD88 expression in CD11c + CD11b + cell compartment is required to sense those species (or other microorganisms that have similar colitis-inducing properties) to trigger inflammatory response in the colon. One question that arises from our data is the cell type responsible for secreting IL-10 and suppressing inflammatory responses in the colon. IL-10 secretion from Tregs has an essential role in maintaining homeostasis in the intestinal mucosa [20] . In addition to Tregs, IL-10 is produced by local MNPs. Previous studies have demonstrated that the two CX 3 CR1 + F4/80 + CD11b + non-migratory macrophage subsets, CD11c − (MP1) and CD11c + (MP2), spontaneously secrete IL-10, even in response to TLR agonists [9] , [10] . These macrophages are thought to be anti-inflammatory, as they actively suppress IL-12 p35 and IL-23 p19 production from colonic lamina propria MNP subsets under non-inflammatory conditions in vivo [9] . Spontaneous IL-10 secretion by these macrophages depends on the presence of commensal flora, but is independent of MyD88 (ref. 9 ). We also observed IL-10 mRNA expression from MP1 CD11c − macrophages (P3) and the P2 population that contains MP2 CD11c + macrophages ( Fig. 5 ). Taken together, these results suggest that IL-10 secretion that normally suppresses inflammatory responses likely comes from Tregs and the immunoregulatory macrophages. It is interesting to note that by genetic ablation of IL-10, these colonic macrophages become highly pathogenic by secreting cytokines that promote Th17 differentiation. Our data also begin to uncover the nature of the colitogenic MNP populations in the colon. On the basis of our observations, we propose a two-step model of colitis progression in IL-10 −/− mice. In the first step, P2 MNPs sense intestinal microbiota and induce proinflammatory cytokines in a MyD88-dependent manner. This is followed by a second step in which inflammatory monocytes are recruited, giving rise to a large number of P3 macrophages capable of secreting more inflammatory cytokines and driving colitic Th17 responses. Evidence for this model comes from our results that in CD11c–MyD88/IL-10 KO mice lacking MyD88 in P1 and P2 but not in P3 population, colitis progression is completely halted, indicating that P2-dependent sensing of microbiota provides a crucial initiating signal and that MyD88 signalling in the P3 population alone is not sufficient to promote colitis. The second line of evidence comes from our observation that P3 macrophages are robustly recruited to the colitic tissue, which outnumber P1 or P2 cells by about 4.3- and 2.2-folds respectively ( Fig. 6b ), suggesting that the inflammatory P3 cells contribute to intestinal inflammation at later stages of colitis. Because of the lack of a mouse system in which MyD88 can be selectively deleted from the P3 cells, it is currently not possible to provide definitive evidence for this hypothesis. The next question that follows is which of the P2 MNP subsets contribute to colitogenesis. We showed that in the IL-10 −/− mice, P2 and P3, but not P1, population upregulate expression of IL-1β, IL-23 p19 and IL-6, and induce Th17 differentiation ex vivo ( Fig. 6 ). These results are highly consistent with a recently published report by Kelsall and colleagues [9] , in which MP1 and MP2 macrophages and CD11b + DC subsets (CD103 − CD11b + and CD103 + CD11b + ), but not the CD103 + CD11b − DCs, upregulated mRNA expression of p35 and p19 in IL-10 −/− mice. Taken together, the P2 subsets that are likely responsible for initiating colitis are the collection of all three MNP types, CD11c + macrophages (MP2), CD103 − CD11b + DCs and CD103 + CD11b + DCs. Inflammatory diseases, once initiated, are often exacerbated by an amplification loop. As discussed above, the amplifier in the IL-10 −/− colitis appears to be the P3 macrophages. Thus, we observed a most dramatic increase in the number of P3 CD11c − macrophages (MP1), which exhibited a highly proinflammatory signature and a Th17-inducing phenotype. Consistent with this finding is a recent report, which showed that intestinal MP1 macrophages (CD11b + CD11c − ) secrete IL-1β in a MyD88-dependent manner and promote Th17 differentiation upon sensing of microbiota in the absence of inflammation [27] . We also observed significant expression of IL-1β in P3 macrophages at steady state, although the level was less than the P2 population ( Fig. 5 ). Collectively, the P3 macrophages are constitutively able to induce IL-1β responses in the gut [27] , but are also recruited to the inflamed colon and amplify colitis in IL-10 −/− mice. However, this may not be universal to all chronic colitis models, as CD103 − CD11b + DCs, but not P3 macrophages, were found to differentiate from circulating inflammatory monocytes, predominate the colon and drive both Th1 and Th17 responses in the T-cell transfer colitis model [9] . Although IL10 −/− and most other models of colitis depend on the presence of 'commensal' bacteria, different components of microbiota are not equivalent in terms of their ability to cause the disease. Indeed, it is increasingly recognized that colitis development is dependent on the presence of 'triggering' bacteria, sometimes also referred to as 'pathobionts' [38] , [39] . It is the presence or absence and the relative abundance of triggering bacteria that determines the timing of onset of colitis and affects the variability in colitis susceptibility in different animal facilities. The bacterial species capable of triggering colitis development in IL10 −/− mice (for example, Helicobacter spp. ) are normally harmless in unmanipulated WT animals. And yet, these animals do mount immune responses to intestinal pathogens. Thus, IL-10 appears to suppress the unwanted immune responses against otherwise harmless bacteria, yet permits the immune response against bacterial pathogens. How this distinction is made by the immune system is unclear, but one possibility is that sensing of pathogen-specific behaviours, such as invasion or production of pore-forming toxins, maybe linked with downregulation of IL-10 production, thus permitting pathogen-specific immune responses. It should also be noted that both commensal and pathogenic bacteria can induce immune responses, but these responses are qualitatively and quantitatively different. It is well known, for example, that the mammalian host generates carefully orchestrated immune responses to commensal bacteria, such as localized sIgA and anti-microbial peptide production [40] , [41] . Such immune responses are likely important to manage the location, composition and density of intestinal bacteria [41] . Importantly, these responses have low tissue-damage potential and, therefore, their constitutive engagement is well tolerated by the host. These responses, however, can be insufficient to suppress the growth or invasion of pathogenic bacteria, which require a far more aggressive immune response, such as Th17- and Th1-mediated response, which is also associated with immunopathology. It is these latter types of immune responses that appear to be suppressed by IL-10 and unleashed in its absence. Activation of these responses, however, still requires the presence of triggering bacteria in the intestines. Interestingly, deletion of A20, a potent negative regulator of the TLR signalling, results in lethal inflammation that is triggered by commensal bacteria and is dependent on MyD88 (ref. 42 ). Thus, the outcome of IL-10 and A20 deletion differs in severity and illustrates non-redundant nature of anti-inflammatory mechanisms. In summary, our study demonstrated a key role for microbiota sensing by colonic MNPs in colitis development in IL-10 −/− mice. Although human genome-wide association studies reveal key inflammatory genes being linked to IBD [43] , treatment options for IBD are limited. One of the key questions in this field relates to the initiation signal that leads to the onset of colitis. Our study provides a clue to the initiating events that underlie disease pathogenesis when the regulatory circuit is dysfunctional. In addition to host genetic lesions, dysbiosis of intestinal microbiota can result in spontaneous transmissible colitis [44] . Defining key anti-inflammatory and proinflammatory circuits that govern our host–microbiota relationship could open promising therapeutic approaches to treating human IBD. Mice A brief summary of the generation of the conditional allele of MyD88 (MGI: 108005) has been published previously [45] , and the detail will be described elsewhere. MyD88 FLOX , MyD88 −/− , IL10 −/− , Villin–Cre, LysM–Cre, CD11c–Cre [14] , WT C57BL/6, Rosa-STOP FLOX EYFP and CX3CR1 gfp mice were bred and maintained under specific pathogen-free conditions at the animal facility of the Yale University School of Medicine. To generate MyD88 conditional KO mice on an IL10 −/− background, MyD88 FL/FL mice were crossed to IL10 −/− and further crossed to Villin–Cre, CD11c–Cre mice. For the study of LysM–MyD88/IL-10 KO mice, MyD88 FL/FL were first crossed to MyD88 −/− mice to generate MyD88 FL/− mice, and then crossed to LysM–Cre mice. Accordingly, both MyD88 FL/− , LysM–Cre, IL-10 −/− and MyD88 FL/FL , LysM–Cre, IL-10 −/− are included as LysM–Cre conditional KO mice (described as LysM–MyD88/ IL-10 KO mice) in this study. Mice were screened for Helicobacter spp . by PCR and 16S rRNA sequences. H. typhlonicus , H. Hepaticus , H. ganmani and H. rodentium were detected in our colony. Studies were approved by the Institutional Animal Care and Use Committee of Yale University. Colonic lamina propria cell preparation and flow cytometry Colons were excised and mesentery was carefully cleaned. Tissue was opened longitudinally, washed of intestinal contents and then was cut into two to three pieces. Tissue was then transferred into 50 ml conical tubes and shaken in PBS containing 2% FCS and 5 mM EDTA for 20–30 min at 37 o C to remove intestinal epithelial cells. To further remove residual epithelial cells, colon tissues were placed in Petri dish and extensively washed in PBS several times using forceps until the supernatants become clear. The remaining tissue was transferred to new 50 ml tubes and digested in PBS containing 2% FCS, 1 unit ml −1 of type VIII collagenase (Sigma-Aldrich) and 10 μg ml −1 of DNase I (Roche) with constant shaking for 60 min at 37 o C. The cells were filtered through a 70-μm cell strainer and washed in PBS two times. Cells were stained with a combination of anti-CD11c (clone HL3), anti-CD11b (clone M170), anti-Siglec-F (clone E50-2440), anti-CD103 (clone M290), anti-CD86 (GL-1), anti-I-A/I-E (M5/114.15.2), anti-DEC205 (205yekta), anti-F4/80 (clone BM8), anti-CD4 (clone L3T4) and anti-Foxp3 (clone FJK-16s) after blockade of Fc receptors. Flow cytometry was performed on a LSR II (BD Biosciences). For some experiments, cells were further sorted on a Moflo (DakoCytomation) or iCyte Reflection (Sony), and were used as lamina propria leukocytes in assays. Histological scoring Colons were excised and divided into three equal segments to be named proximal, middle and distal colon. Middle colon tissue was fixed in with Bouin's fixative (Sigma-Aldrich) for 30 min, paraffin embedded, sectioned and stained with haematoxylin and eosin. Sections were analysed and scored for the levels of inflammation by a pathologist in a blind manner. The score was evaluated on the basis of epithelial hyperplasia, mononuclear infiltrate and polymorphonuclear infiltrate (0=none; 1=mild; 2=moderate; 3=severe). Colon tissue culture Segment (1 cm) of proximal colon were excised and washed in cold PBS supplemented with penicillin and streptomycin. Tissue was placed in 24-well plate with 1 ml of serum-free RPMI 1640 medium supplemented with penicillin and streptomycin. After 24 h, supernatants were collected as samples. MLN cell culture MLNs were excised and grinded by sterile frosted slides and then filtered through a 70-μm cell strainer to make single cell suspension. Cells (2×10 6 ) were plated into 24-well plates and incubated in the presence of plate-bound anti-CD3ε (1 μg ml −1 ; clone 145–2C11) in 1 ml of complete medium (RPMI 1640 containing 10% FCS, 100 U ml −1 penicillin–streptomycin, 2 mM L -glutamine, 1 mM sodium pyruvate, 10 mM HEPES and 50 μM β-mercaptoethanol). After 48 h, supernatants were collected and cytokines were measured by enzyme linked immunosorbant assay (ELISA). Colonic lamina propria cell culture Bulk colonic lamina propria cells obtained after collagenase treatment described in 'Colonic lamina propria cell preparation' were subjected to density-gradient centrifugation in 44 to 65% Percoll (GE Healthcare). The cells at the interface were collected and washed in PBS two times. Cells were plated into 24-well plates at the concentration of 7.5×10 5 cells ml −1 and incubated in the presence of plate-bound anti-CD3ε (1 μg ml −1 ; clone 145–2C11) for 48 h. The supernatants were collected and cytokines were measured by ELISA assay. Cytokine quantification by ELISA assay Paired antibodies (anti-mouse purified and biotinylated; IL-12 p40; clone C17.6 and C17.8, and IL-17A; clone eBio17CK15A5 and eBio17B7, and IFN-γ; clone XMG1.2 and clone R4-6A2, respectively) and recombinant standards for IL-12 p40, IL-17A and IFN-γ were used to quantify factors present in supernatants of colon tissue, MLNs and lamina propria cell and T-cell cultures. Isolation of RNA and quantitative RT–PCR For isolation of colon tissue mRNA, the tissue was homogenized in RNA-Bee (TEL-TEST, Inc.) and total RNA was isolated according to manufacturer's instructions. For FACS-sorted cell mRNA isolation, RNeasy kit (Qiagen) was used. Complementary DNAs were prepared using SMART MMLV reverse transcriptase (Clontech) and used for PCR with SYBR Green reagents (Qiagen or Quanta Bioscience) on a Stratagene MX3000 bioanalyser. The abundance of mRNA of target genes was normalized to hypoxanthine guanine phosphoribosyl transferase expression. Sequences of the primers used in this study are shown in the Supplementary Table S1 . In vitro T-cell stimulation Naive T cells from the spleens of C57BL/6 were purified by magnetic sorting with mouse anti-CD4 beads (clone L3T4, Miltenyi Biotec). T cells (1×10 5 ) were co-cultured with 2×10 4 purified colonic lamina propria leukocytes in 200 μl complete medium (RPMI 1640 containing 10% FCS, 100 U ml −1 penicillin–streptomycin, 2 mM L -glutamine, 1 mM sodium pyruvate, 10 mM HEPES and 50 μM β-mercaptoethanol) in the presence of anti-CD3ε antibody in 96-well plates. After 72 h incubation, supernatants were collected as samples. Endoscopic analysis Colonoscopy was performed in a blinded fashion for colitis scoring via the Coloview System (Karl Storz, Germany) [21] . In brief, colitis scoring was based on granularity of mucosal surface, stool consistence, vascular pattern, translucency of the colon and fibrin visibility (0–3 points for each). Statistical analysis Statistical significance was evaluated with an unpaired two-tailed Student's t -test. A P -value of less than 0.05 was considered significant (Prism; GraphPad Software, Inc.). How to cite this article: Hoshi, N. et al . MyD88 signalling in colonic mononuclear phagocytes drives colitis in IL-10-deficient mice. Nat. Commun. 3:1120 doi: 10.1038/ncomms2113 (2012).